Reply to: The stress-inducible ER chaperone GRP78/BiP is upregulated during SARS-CoV-2 infection and acts as a pro-viral protein 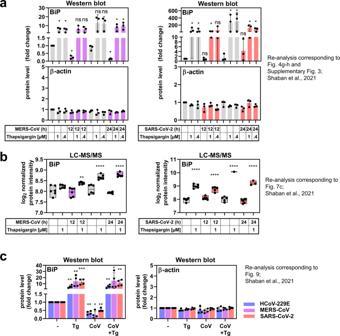Fig. 1: Additional quantifications of changes in BiP levels from MERS-CoV or SARS-CoV-2-infected cells in the presence or absence of thapsigargin (Tg) reported by Shaban et al.1. aGraphs with split Y-axes showing the quantification of BiP and β-actin protein bands in HuH7 cells infected with MERS-CoV (MOI of 0.5) or Vero E6 cells infected with SARS-CoV-2 (MOI of 0.5) for 12 h or 24 h as previously presented in Supplementary Fig. 3 of Shaban et al.,1. Data points represent three biologically independent experiments. Representative immunoblots are provided in Fig. 4 g (MERS-CoV) and Fig. 4 h (SARS-CoV-2) of Shaban et al.,1. BiP levels were quantified relative to the untreated control. Bar graphs show means ± s.d.; asterisks indicate significant changes (*p≤ 0.05) obtained by two-tailed ratio-pairedt-tests; ns indicates non-significant changes.bNormalized protein intensity values of BiP expression were determined by label-free LC-MS/MS-based quantification of tryptic peptides derived from total cell extracts of uninfected HuH7 cells (−), cells infected with MERS-CoV (MOI of 3) for 12 h or 24 h (left graphs), or Vero E6 cells infected with SARS-CoV-2 (MOI of 3) for 12 h or 24 h (right graphs), in the presence or absence of thapsigargin (1 µM). At least 53 (Huh7 cells) or 78 (Vero E6 cells) unique peptides were obtained, representating a sequence coverage of BiP ranging from 60.1 to 69.6%. Raw data can be retrieved using the following link: 10.6019/PXD021222. Floating bars show minimum to maximum values and means. Data points represent two biological and three technical replicates. Asterisks indicatepvalues (*p≤ 0.05, **p≤ 0.01, ***p≤ 0.001, ****p≤ 0.0001) obtained by ordinary one-way ANOVA.cGraphs with splitY-axes showing the quantification of BiP and β-actin protein bands in HuH7 cells infected with HCoV-229E (MOI of 3), MERS-CoV (MOI of 3) or Vero E6 cells infected with SARS-CoV-2 (MOI of 3) for 24 h as previously presented in Fig. 9b of Shaban et al.,1. Data points represent four biologically independent experiments. Representative immunoblots are shown in Fig. 9a of Shaban et al.,1. BiP levels were quantified relative to the untreated control. Bar graphs show means ± s.d.; asterisks indicate significant changes (*p≤ 0.05, **p≤ 0.01, ***p≤ 0.001) obtained by two-tailed ratio-pairedt-tests; ns indicates non-significant changes. Cells and viruses Viruses and cell sources between the two studies differ. Specifically, in the study by Shaban et al. [1] , the following cell lines and virus strains were used: HuH7 human hepatoma cells (Japanese Collection of Research Bioresources cell bank), which were maintained in Dulbecco’s modified Eagle’s medium (DMEM) complemented with 10% filtrated bovine serum (FBS Good Forte; PAN Biotech, Cat No. P40-47500), 2 mM L-glutamine, 100 U/ml penicillin and 100 μg/ml streptomycin and Vero E6 African green monkey kidney epithelial cells (ATCC CRL-1586), which were grown in DMEM, 10% FBS, 100 U/ml penicillin, and 100 μg/ml streptomycin. Genome sequences of coronavirus strains were as follows: HCoV-229E (NCBI accession number AF304460.1, NCBI reference sequence NC_002645.1), MERS-CoV (NCBI accession number JX869059, NCBI reference sequence NC_01984 3.3). SARS-CoV-2 (NCBI Short Read Archive repository under bioproject PRJNA658242 (SRA accession number SRX9907172 and SRX8975039). MERS-CoV and SARS-CoV-2 were kindly provided by Christian Drosten. All further details are available in Shaban et al. [1] . Protein analyses Cell lysis, protein extraction, Western blotting and mass spectrometry-based proteomics analyses are described in detail in Shaban et al. [1] . Statistics, quantification, and reproducibility Quantification of data and statistical parameters were calculated using GraphPad Prism 5.0, 8.4.3, or 9.4.1, Perseus (versions 1.6.10.50 (MERS-CoV) or 1.6.14 (SARS-CoV-2)), ImageLab (versions 5.2.1 or 6.0.1) and Microsoft Excel 2016. Further details are given in Shaban et al. [1] . Reporting summary Further information on research design is available in the Nature Research Reporting Summary linked to this article.